A ladder polysilane as a template for folding palladium nanosheets Although discrete nano-sized compounds consisting of a monolayer sheet of multiple atoms have attracted much attention, monolayer transition metal nanosheets are difficult to access. Here we report a template synthesis of the folding metal nanosheet ( 2 ) consisting of 11 palladium atoms by treatment of a ladder polysilane, decaisopropylbicyclo[2.2.0]hexasilane ( 1 ), with Pd(CN t Bu) 2 . Crystallographic analysis reveals that the compound is composed of two monolayer Pd 7 sheets sharing three palladium atoms at the junction. Each Pd atom is stabilized by Pd–Si σ-bonds, Pd–Pd bonds and coordination of isocyanides. Ligand exchange of 2 from CN t Bu to CN(2,4,6-Me 3 -C 6 H 2 ) is accompanied by structural rearrangement, leading to the formation of another folding Pd 11 nanosheet ( 3 ) consisting of two edge-sharing Pd 7 sheets. The shapes of the Pd 7 sheets as well as the dihedral angle between the two Pd 7 sheets are dependent on the substituent of the isocyanide ligand. The isolation of graphene from graphite, typically by scratching away multilayers of graphite, has made it possible to access a new form of carbon with nanosheet structures [1] , [2] , [3] , [4] . Several metal oxides and sulphides having multilayered structures also form nanosheets by peeling off their monolayers [5] . These nanosheets show profoundly different physical properties from their precursors, eliciting much interest in nanoscience. These nanosheets suggest the possible preparation of transition metal nanosheets; however, the lack of precursors to which to apply mechanical separation suitable for isolation of monolayers prevents easy access to these compounds. The synthesis of relatively small transition metal nanosheets has attained some success in organometallic and inorganic chemistry [6] , [7] , [8] , [9] . Among them, a novel methodology to synthesize Pd 3 to Pd 5 nanosheets was developed by Murahashi et al. [10] , [11] , [12] , [13] , [14] , [15] , [16] using (poly)cyclic aromatic hydrocarbons as a template for the arrangement of Pd atoms in a two-dimensional sheet structure. The sandwich compound, [Pd 5 (naphthacene) 2 ] 2+ , is the largest palladium nanosheet reported to date [10] . Success of this template synthesis of transition metal nanosheets suggests a strategy to access new nanosheets using templates that force the metals into a planar arrangement owing to metal–metal bonding interactions. In this paper, we report a ladder polysilane, decaisopropylbicyclo[2.2.0]hexasilane ( 1 ) [17] , [18] , [19] , [20] , that serves as a template for two Pd 11 clusters, 2 and 3 , which are considered to be folding metal nanosheets having two planar Pd 7 units. The array of Pd and Si atoms and the dihedral angle of the two Pd 7 sheets are dependent on the substituent of the isocyanide ligand. Synthesis of folding Pd 11 nanosheet 2 Insertion of a Pd(CNR) 2 species between a Si–Si bond of oligosilanes to give complexes of the type (RNC) 2 Pd(SiR 3 ) 2 has been investigated extensively by Ito and coworkers [21] , [22] . These complexes serve as intermediates for catalytic transformations of oligosilanes. However, only a few cyclic oligosilanes were subjected to the study, and they were reportedly less reactive than their linear analogues even at elevated temperatures. Our new discovery, a ladder polysilane having seven Si–Si bonds in a molecule, decaisopropylbicyclo[2.2.0]hexasilane ( 1 ), is highly reactive towards Pd(CN t Bu) 2 ( t Bu= t -butyl), and the reaction unexpectedly leads to the formation of the Pd 11 cluster 2 . As shown in Fig. 1 , treatment of 1 with 11 equivalents of Pd(CN t Bu) 2 in toluene at room temperature resulted in complete consumption of 1 after 18 h. The product 2 was isolated as dark green crystals suitable for crystallography in 65% yield by recrystallization from toluene/pentane at −35 °C. The molecular structure of 2 ( vide infra ) suggests that oxidative addition of Pd(CN t Bu) 2 moieties into seven Si–Si bonds in 1 explains the origin of seven Pd atoms in 2 , and an additional four Pd atoms participate in the construction of the folding nanosheet structure. No intermediary species were visible in the reaction from 1 to 2 . Indeed, treatment of 1 with seven equivalents of Pd(CN t Bu) 2 resulted in exclusive formation of 2 (65%) with recovery of 1 (35%). 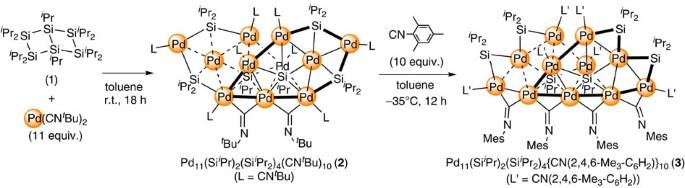Figure 1: Synthesis of2and3. Synthesis of2by using a ladder polysilane (1) as the template, and synthesis of3by ligand exchange and skeletal rearrangement. r.t., room temperature. Figure 1: Synthesis of 2 and 3 . Synthesis of 2 by using a ladder polysilane ( 1 ) as the template, and synthesis of 3 by ligand exchange and skeletal rearrangement. r.t., room temperature. Full size image Molecular structure of 2 The molecular structure of 2 is depicted in Fig. 2a and Supplementary Figs S1 and S2 . The molecular structure of Pd 11 cluster 2 can be regarded as one large folding nanosheet containing eleven palladium atoms or two small nanosheets (Pd 7 sheet I and Pd 7 sheet II in Fig. 2a ) consisting of seven palladium atoms each, sharing three palladium atoms at the junction. The dihedral angle between sheets I and II is 37.7° ( Fig. 2c and Supplementary Fig. S3 ). Each Pd 7 sheet contains two silylene moieties, Si i Pr 2 ( i Pr= i -propyl), which are located in the plane of the Pd 7 sheet, whereas one silylyne group, Si i Pr, is located out of the plane as described later in more detail. Four palladium atoms at the edge of the Pd 7 sheet are bonded to the terminal isocyanide ligands. Three linearly assembled Pd atoms, Pd(5), Pd(6) and Pd(7), lie on the junction ( Fig. 2d ), and two CN t Bu ligands bridge the Pd(5)–Pd(6) and Pd(6)–Pd(7) bonds to enhance the Pd–Pd interactions. 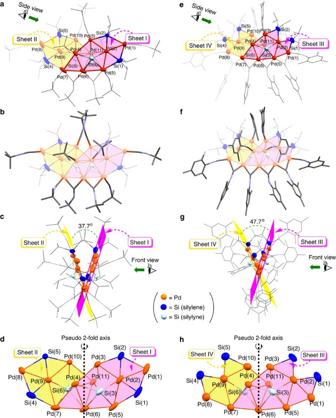Figure 2: Molecular structures of2and3. (a) Front view of2(Pd11Si6core was emphasized). (b) Front view of2(CNtBu ligands were emphasized). (c) Side view of2. (d) Array of Pd and Si atoms of2. (e) Front view of3(Pd11Si6core was emphasized). (f) Front view of3(CN(2,4,6-Me3-C6H2) ligands were emphasized). (g) Side view of3. (h) Array of Pd and Si atoms of3.Probability ellipsoids shown at 50%. Figure 2: Molecular structures of 2 and 3 . ( a ) Front view of 2 (Pd 11 Si 6 core was emphasized). ( b ) Front view of 2 (CN t Bu ligands were emphasized). ( c ) Side view of 2 . ( d ) Array of Pd and Si atoms of 2 . ( e ) Front view of 3 (Pd 11 Si 6 core was emphasized). ( f ) Front view of 3 (CN(2,4,6-Me 3 -C 6 H 2 ) ligands were emphasized). ( g ) Side view of 3 . ( h ) Array of Pd and Si atoms of 3. Probability ellipsoids shown at 50%. Full size image Synthesis of another folding Pd 11 nanosheet 3 To our surprise, the CN t Bu ligands were reactive towards ligand exchange by other isocyanide ligands, for example, CN(2,4,6-Me 3 -C 6 H 2 ). Treatment of 2 with ten equivalents of CN(2,4,6-Me 3 -C 6 H 2 ) in toluene at −35 °C for 12 h resulted in quantitative displacement of all of the CN t Bu ligands with CN(2,4,6-Me 3 -C 6 H 2 ) to produce the new Pd 11 cluster 3 in 55% yield after recrystallization from ether ( Fig. 1 ). X-ray structure analysis revealed that compound 3 also has a folding Pd 11 nanosheet structure similar to 2 ( Fig. 2e and Supplementary Figs S4 and S5 ). However, the dihedral angle (47.7°) between the two Pd 7 sheets ( Fig. 2g and Supplementary Fig. S6 ) is significantly different from that in 2 . Similar to 2 , each Pd 7 nanosheet is supported by two silylene units in the plane and one silylyne moiety out of the plane; however, the array of Pd and Si atoms is different from that in 2 ( vide infra ). Three palladium atoms at the edge of the Pd 7 sheet are bonded to terminal isocyanide ligands, whereas five Pd atoms, Pd(1), Pd(5), Pd(6), Pd(7) and Pd(8), aligning in a slightly curved line are bound to four bridging isocyanide ligands ( Fig. 2h ). Detailed molecular structures of 2 and 3 Several unique points should be noted in the molecular structures of 2 and 3 . First, both 2 and 3 consist of eleven palladium atoms, six organosilyl moieties and ten isocyanide ligands with formula Pd 11 (Si i Pr 2 ) 4 (Si i Pr) 2 (CNR) 10 . Second, both 2 and 3 have a pseudo twofold axis passing through the Pd(6) atom and the midpoint of the Pd(4) and Pd(11) atoms as shown in Fig. 2d . Third, each half, that is, Pd 7 sheets I and II in 2 and Pd 7 sheets III and IV in 3 , consists of a Pd 7 (Si i Pr 2 ) 2 (Si i Pr) subunit. Owing to the pseudo- C 2 -symmetric structures of 2 and 3 , the Pd 7 sheets I and II in 2 or the Pd 7 sheets III and IV in 3 can be regarded as structurally equivalent. In fact, all of the Pd–Pd, Pd–Si and Pd–C distances and related bond angles in I or III are comparable to those of II or IV. In Fig. 3 are depicted the array of Pd and Si atoms in the Pd 7 sheet I (a–d) and the Pd 7 sheet III (e and f). For both Pd 7 sheets I and III, the seven palladium and two silicon atoms of the Pd 7 (Si i Pr 2 ) 2 (Si i Pr) subunit are located in the same plane to form the planar Pd 7 Si 2 nanosheet structure. The deviations of all atoms from the plane defined by the Pd 7 Si 2 nanosheet are within the range of ca. 0.00–0.35 Å for Pd 7 sheet I ( Supplementary Fig. S7 ). The deviation is somewhat larger in Pd 7 sheet III (ca. 0.08–0.40 Å) ( Supplementary Fig. S8 ). The remaining silicon atom derived from the silylyne moiety (Si(3) in both I and III) is located below the Pd 7 Si 2 plane. This Si atom may act as the anchor to reinforce the Pd 7 Si 2 nanosheet structure. 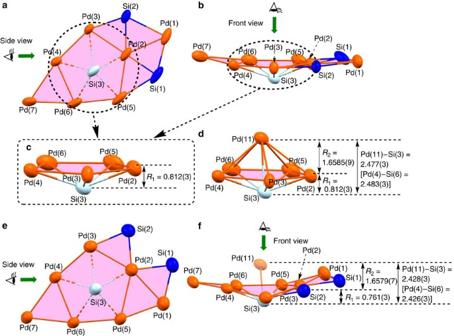Figure 3: Core-atom representations of the solid-state structures of2and3. (a) Front view of the Sheet I. (b) Side view of the Sheet I. (c) Side view of the pentagonal pyramidal subunit of the Sheet I. (d) Side view of one of the pentagonal bipyramidal substructure of2. (e) Front view of the Sheet III. (f) Side view of the Sheet III. Probability ellipsoids shown at 50%. Figure 3: Core-atom representations of the solid-state structures of 2 and 3. ( a ) Front view of the Sheet I. ( b ) Side view of the Sheet I. ( c ) Side view of the pentagonal pyramidal subunit of the Sheet I. ( d ) Side view of one of the pentagonal bipyramidal substructure of 2 . ( e ) Front view of the Sheet III. ( f ) Side view of the Sheet III. Probability ellipsoids shown at 50%. Full size image A characteristic feature of Pd 7 sheet I is that there is a planar pentagonal Pd 5 unit consisting of Pd(2), Pd(3), Pd(4), Pd(5) and Pd(6), and the Si(3) atom of the silylyne moiety is located below this pentagonal plane by 0.812(3) Å ( Fig. 3c ). One of the other two palladium atoms of Pd 7 sheet I, that is, Pd(7) in Fig. 3a , completes the triangular substructure along with Pd(4) and Pd(6). The same characteristic arrangement of Pd and Si atoms is also seen in Pd 7 sheet III. The orientation of the remaining Pd atom (Pd(1) in Fig. 3a ) is different between Pd 7 sheets I and III: the Pd(1) atom in I is located at the edge of the Pd 7 Si 2 plane to bisect the Si(1)–Pd(2)–Si(2) angle, whereas that in III is arranged next to the Pd(5)–Pd(6)–Pd(7) junction to form a bridge over the Pd(2) and Pd(5) atoms. The Pd–Pd bond distances in Pd 7 sheets I and III are within the range of 2.674(2)–2.9998(11) Å for I ( Supplementary Fig. S9 ) and 2.6168(12)–2.8779(12) Å for III ( Supplementary Fig. S10 ), which are comparable to those found in previously reported polynuclear palladium clusters, including planar triangular or tetranuclear clusters [23] , [24] , [25] , [26] , [27] , [28] , [29] , [30] , [31] . Two Si atoms derived from the silylene moiety (Si(1) and Si(2)) are located on the edge of Pd 7 sheets I and III ( Fig. 3a ). It should be mentioned that the coordination number of these silicon atoms is different in Pd 7 sheets I and III. The coordination geometry in sheet I is pentacoordinate to form the distorted trigonal bipyramidal structure involving two i Pr groups and three Pd atoms, whereas sheet III contains tetracoordinated silicon atoms connected to two i Pr groups and two Pd atoms. As mentioned above, there are planar pentagonal Pd 5 subunits in Pd 7 sheets I and III. One silicon atom (Si(3)) located below this plane is connected to these five Pd atoms to form the pentagonal pyramidal structure ( Fig. 3c and Supplementary Figs S11 and S12 ). The Si(3) atom in sheet I is out of the Pd 5 plane by 0.812(3) Å, whereas the position of the Si(3) atom in sheet III deviates from the plane by 0.761(3) Å ( Fig. 3f ). It is worthwhile to point out that there is an interplane bonding interaction between Si(3) in Pd 7 sheet I and Pd(11) in Pd 7 sheet II ( Fig. 3d ); this explains the dihedral angle between Pd 7 sheets I and II of 37.7°. The Si(3)–Pd(11) bond distance of 2.477(3) Å is longer than that found in common Pd–Si complexes (around 2.3–2.4 Å) [32] , [33] , but shorter than several Pd–Si bonds seen in Osakada’s planar Pd 4 Si 3 cluster (2.5052(8)–2.5456(7) Å) [28] . Similarly, the interplane bonding of Si(3) in sheet III and Pd(11) in sheet IV is the origin of the dihedral angle of 47.7°. As a consequence of the interplane bonding interaction, a pentagonal bipyramidal substructure was formed in the Pd 6 Si unit, and Si(3) is bound to one isopropyl group and six palladium atoms to make the heptacoordinate silicon centre. Silicon atoms stabilized by six metal atoms (μ 6 -coordination) are rarely found in the literature [34] , [35] . A conceptual scheme to construct the folding Pd 11 (Si i Pr 2 ) 4 (Si i Pr) 2 (CNR) 10 nanosheet structure is depicted in Fig. 4 using compound 2 as a representative example. First, the Pd 7 (Si i Pr 2 ) 2 (Si i Pr)(CNR) 5 subunits, namely Pd 7 nanosheets I and II, were formed with the aid of the bridging silylyne moiety; then sheets I and II were connected to each other to form the planar Pd 11 (Si i Pr 2 ) 4 nanosheet. Bending this planar nanosheet along the linear Pd(5)–Pd(6)–Pd(7) junction afforded the folding Pd 11 (Si i Pr 2 ) 4 nanosheet having a pseudo- C 2 -symmetric structure. 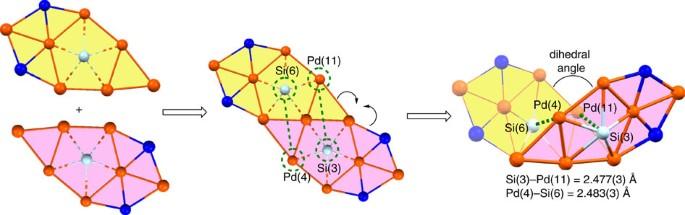Figure 4: The conceptual scheme to construct the folding nanosheet. Template synthesis of the folding Pd11nanosheet with the aid of bridging silylene and silylyne moieties. Figure 4: The conceptual scheme to construct the folding nanosheet. Template synthesis of the folding Pd 11 nanosheet with the aid of bridging silylene and silylyne moieties. Full size image It is of interest that the dihedral angles of the two Pd 7 Si 2 sheets are different in 2 and 3 (37.7° ( 2 ) and 47.7° ( 3 )). In both 2 and 3 , the folding structure is induced by the interaction of Pd(11)–Si(3) and Pd(4)–Si(6) as described above. The bond lengths of Pd(11)–Si(3) and Pd(4)–Si(6) in 2 (2.477(3) and 2.483(3) Å) are slightly longer than those in 3 (2.428(3) and 2.426(3) Å). This seems inconsistent with the smaller dihedral angle of 2 than that of 3 . This contradiction is explained by the larger deviation of the silylyne atoms (Si(3) or Si(6)) from the planar Pd 7 (Si i Pr 2 ) 2 subunit in 2 ( R 1 =0.812(3) Å for 2 in Fig. 3d ) than that in 3 ( R 1 =0.761(3) Å in Fig. 3f ). The shorter R 1 contributes to increase the dihedral angle, whereas the shorter Pd(11)–Si(3) or Pd(4)–Si(6) distance takes part in decreasing it. The large dihedral angle of 3 indicates that the former is more effective in determining the dihedral angle. Molecular structures of 2 and 3 in solution The 1 H and 13 C{ 1 H} NMR spectra of 2 are consistent with those expected from their C 2 -symmetric molecular structures ( Supplementary Figs S13 and S14 ). The 29 Si{ 1 H} NMR spectrum of 2 displayed three sharp signals ( Supplementary Fig. S15 ), the significant downfield shifts of which are characteristic of bridging silylene ( δ 191.85, 226.63) and silylyne ( δ 327.54) moieties [36] . The electrospray ionization mass spectrometry (ESI-MS) spectrum of 2 also supports this, giving two peaks at m/z 2519 and 2602, which are assignable to [ 2 -CN t Bu]+H + and [ 2 ]+H + , respectively ( Supplementary Figs S16 and S17 ). These indicate that the C 2 -symmetric Pd 11 Si 6 units in 2 were maintained in solution. Owing to their thermal instability in solution, the detection of signals in 29 Si{ 1 H} NMR and ESI-MS of 3 was difficult. However, 1 H and 13 C{ 1 H} NMR spectra of 3 suggest that the structure in solution is identical with that seen in the solid state ( Supplementary Figs S18 and S19 ). Variable temperature 1 H NMR studies showed dynamic behaviour due to site exchange of the isocyanide ligand in 2 but not in 3 ( Supplementary Fig. S20 ). To the best of our knowledge, 2 and 3 are the only examples of discrete folding metal nanosheets unequivocally characterized by crystallography and spectroscopy. These Pd 7 subunits are the largest planar clusters reported in the literature. More than 40 palladium clusters that are larger than pentanuclear are found in the Cambridge Structural Database (ConQuest version 1.14, February 2013). Most of them were synthesized by tedious multistep procedures in low to medium yields. None of them has a two-dimensional nanosheet structure except Murahashi’s Pd 5 cluster described above. Therefore, it is remarkable that a folding Pd 11 Si 4 nanosheet 2 is synthesized in high yield in a single step using the ladder polysilane 1 as a template, and another folding Pd 11 Si 4 nanosheet 3 is formed by exchange of all the CN t Bu ligands in 2 to CN(2,4,6-Me 3 -C 6 H 2 ). During the conversion from 2 to 3 , the array of Pd and Si atoms is altered, and the dihedral angle between the two Pd 7 sheets becomes larger. New properties of nano-sized transition metal compounds have attracted attention from a wide array of scientists. Discovery of the ladder polysilane as a template for Pd nanosheets could open the way to synthesize new types of nanometal compounds. Synthesis of materials Manipulation of air- and moisture-sensitive compounds was carried out under dry nitrogen atmosphere using standard Schlenk tube techniques associated with a high-vacuum line or in the M. Braun Unilab N 2 -filled glove box maintained at or below 1 p.p.m. of O 2 and H 2 O. Glassware was dried at 100 °C for 1 h. All commercial reagents were used as received unless otherwise noted. All solvents (toluene, pentane, diethyl ether, toluene-d 8 and C 6 D 6 ) were distilled over Na/benzophenone and vacuum transferred to a storage container before use. Pd(CN t Bu) 2 was synthesized using a published method [22] , [37] . Mesityl isocyanide was prepared according to a modified literature procedure [38] . Decaisopropylbicyclo[2.2.0]hexasilane ( 1 ) was synthesized by the method reported in the literature [18] , [20] . Synthesis of 2 In a 20 ml Schlenk tube, Pd(CN t Bu) 2 (100 mg, 0.37 mmol) was dissolved in toluene (3 ml), and toluene (2 ml) solution of decaisopropylbicyclo[2.2.0]hexasilane ( 1 ) (20 mg, 0.03 mmol) was added at room temperature. The colour of the initial solution gradually became dark green within 6 h. After mixing this dark green solution for 18 h at room temperature, the solvent was removed in vacuo . The remaining crude product was washed with pentane (5 ml × 3), and dissolved in toluene (3 ml). This toluene solution was centrifuged to remove the small amount of insoluble materials. The supernatant was collected, layered with pentane (5 ml) and cooled to −35 °C to afford the dark green crystals of 2 (56 mg, 0.02 mmol, 65%). 1 H NMR (600 MHz, 20 °C, C 6 D 6 ) δ 0.95–1.05 (broad s, 18H), 1.21–1.36 (broad s, 18H), 1.30 (s, 18H), 1.40 (s, 18H), 1.44–1.59 (broad s, 18H), 1.48 (d, J =7.1 Hz, 6H), 1.67 (d, J =7.1 Hz, 6H), 1.78 (d, J =7.1 Hz, 6H), 1.86 (d, J =7.1 Hz, 6H), 1.87 (d, J =7.1 Hz, 6H), 1.90 (d, J =7.1 Hz, 6H), 1.93 (d, J =7.1 Hz, 6H), 1.99 (d, J =7.1 Hz, 6H), 2.14 (d, J =7.1 Hz, 6H), 2.24 (d, J =7.1 Hz, 6H), 2.35–2.47 (m, 10H). 13 C NMR (150 MHz, 20 °C, C 6 D 6 ): δ 23.58, 23.89, 24.18, 24.20, 24.74, 24.91, 25.12, 25.36, 25.84, 26.28, 26.62, 26.70, 26.94, 28.08, 30.14 (broad s), 30.22, 30.31 (broad, s), 30.76, 31.04 (broad s), 31.49, 54.09 (broad s), 54.41, 54.63, 56.41 (broad s), 150.40, 153.81, 155.02 (broad s), 165.92 (broad s) (one C Me 3 and one C =N t Bu) peak are missing presumably owing to the overlapping). 29 Si NMR (119 MHz, 20 °C, C 6 D 6 ): δ 191.85 (s), 226.63 (s), 327.54 (s); IR (KBr pellet): ν N≡C =2026–2202 (broad) cm −1 . ESI-MS (THF, 20 °C): m / z =2519 ([ 2 -CN t Bu]+H + ; 100%) and 2602 ([ 2 ]+H + ; 49%). Anal calcd for C 80 H 160 N 10 Pd 11 Si 6 ; C 36.94, H 6.20, N 5.38; found: C 36.57, H 6.05, N 5.09. Synthesis of 3 In a 20 ml Schlenk tube, Pd 11 (Si i Pr 2 ) 4 (Si i Pr) 2 (CN t Bu) 10 ( 2 ) (50 mg, 0.02 mmol) was dissolved in toluene (3 ml), and toluene (2 ml) solution of mesityl isocyanide (28 mg, 0.19 mmol) was added at −35 °C. After the resulting mixture was stirred for 12 h at −35 °C, the solvent was removed under reduced pressure. The residue was dissolved in pentane (5 ml), and centrifuged to remove the small amount of insoluble materials. The supernatant was collected, and the solvent was evaporated in vacuo . The remaining powder was dissolved in diethyl ether (3 ml), and cooled to −35 °C to afford the dark green crystals of 3 (34 mg, 0.01 mmol, 55%). 1 H NMR (600 MHz, 20 °C, C 6 D 6 ): δ 1.21–1.31 (m, 2H), 1.47 (d, J =7.7 Hz, 6H), 1.53 (d, J =7.1 Hz, 6H), 1.56 (d, J =7.7 Hz, 6H), 1.58 (broad s, 6H), 1.59 (d, J =7.7 Hz, 6H), 1.80 (broad s, 6H), 1.82–1.86 (m, 18H), 1.88 (d, J =7.7 Hz, 6H), 1.89 (s, 12H), 1.90 (s, 6H), 1.99 (s, 6H), 2.03 (d, J =7.1 Hz, 6H), 2.12 (d, J =7.1 Hz, 6H), 2.15 (broad s, 18H,), 2.20 (s, 12H), 2.22 (d, J =7.7 Hz, 6H), 2.50 (s, 12H), 2.56 (s, 12H), 2.90–3.02 (m, 2H). 13 C NMR (150 MHz, 20 °C, C 6 D 6 ): δ 14.29 (broad s), 18.55, 18.82, 19.09, 19.27, 19.92, 20.94, 20.96, 21.08, 21.13 (broad s), 22.04, 22.08, 22.25, 22.51, 22.60, 22.74, 24.16, 24.93, 25.40, 26.19, 27.97, 29.61, 30.19, 34.45, 35.40, 126.80, 128.63, 128.88, 128.90, 129.31, 130.66, 132.06, 132.11, 133.55, 133.65, 133.68, 133.93, 133.99, 134.37, 134.44, 134.48, 134.49, 136.07, 136.97, 165.95, 168.71, 168.75, 173.34, 180.05 (one aromatic peak is missing presumably owing to the overlapping). IR (KBr pellet): ν N≡C =1968–2160 (broad) cm −1 . Anal calcd for C 130 H 180 N 10 Pd 11 Si 6 ; C 48.46, H 5.63, N 4.35; found: C 48.19, H 5.43, N 4.08. X-ray data collection and reduction X-ray crystallography was performed on a Rigaku Saturn CCD area detector with graphite monochromated Mo-Kα radiation ( λ =0.71070A). The data were collected at 123(2) K using ω scan in the θ range of 3.03≤θ≤27.54 deg ( 2 ) and 3.05≤θ≤27.54 deg ( 3 ). The data obtained were processed using Crystal-Clear (Rigaku) on a Pentium computer, and were corrected for Lorentz and polarization effects. The structures were solved by direct methods, and expanded using Fourier techniques. Hydrogen atoms were refined using the riding model. The final cycle of full-matrix least-squares refinement on F 2 was based on 24,780 observed reflections and 975 variable parameters for 2 and 31,308 observed reflections and 1,296 variable parameters for 3 . Neutral atom scattering factors were taken from Cromer and Waber. All calculations were performed using the CrystalStructure crystallographic software package. Two of ten t Bu groups in 2 were observed at two positions with the site occupancy factor of 0.50:0.50, and these t Bu groups were refined isotropically. The disordered pentane solvent was found in the unit cell of 2 . One of the i Pr group of 3 showed the disorder in the crystal. The site occupancy factor of 0.30:0.30:0.40 was determined, and the carbon atoms derived from this i Pr group was refined isotropically. It was found that three mesityl groups of 3 were highly disordered, thus the carbon atoms of them were refined using geometrical restraint. Details of the final refinement are summarized in the Supplementary Table S1 . Accession codes: The X-ray crystallographic coordinates for structures reported in this Article have been deposited at the Cambridge Crystallographic Data Centre (CCDC), under deposition numbers CCDC 924691 and 924692. These data can be obtained free of charge from The Cambridge Crystallographic Data Centre via www.ccdc.cam.ac.uk/data_request/cif . How to cite this article: Sunada, Y. et al. A ladder polysilane as a template for folding palladium nanosheets. Nat. Commun. 4:2014 doi: 10.1038/ncomms3014 (2013).